eQTL mapping identifies insertion- and deletion-specific eQTLs in multiple tissues Genome-wide gene expression quantitative trait loci (eQTL) mapping have been focused on single-nucleotide polymorphisms and have helped interpret findings from diseases mapping studies. The functional effect of structure variants, especially short insertions and deletions (indel) has not been well investigated. Here we impute 1,380,133 indels based on the latest 1,000 Genomes Project panel into three eQTL data sets from multiple tissues. Imputation of indels increased 9.9% power and identifies indel-specific eQTLs for 325 genes. We find introns and vicinities of UTRs are more enriched of indel eQTLs and 3.6 (single-tissue)–9.2%(multi-tissue) of previous identified eSNPs were taggers of eindels. Functional analyses identifies epigenetics marks, gene ontology categories and disease GWAS loci affected by SNPs and indels eQTLs showing tissue-consistent or tissue-specific effects. This study provides new insights into the underlying genetic architecture of gene expression across tissues and new resource to interpret function of diseases and traits associated structure variants. In the past decade, most common single-nucleotide polymorphism (SNP) with allele frequency >5% have been identified and genome-wide association studies (GWAS) have been focusing on these common variants. As of February 2014, 1,785 studies have detected disease susceptibility loci at genome-wide significant level [1] ( www.genome.gov/GWAStudies ). However, discovery has only explained a modest portion of disease risk [2] . The undetected variants could be due to common SNPs but without sufficiently large effect, structure variants such as short insertion and deletion (indel) or low-frequency SNP not covered by genotyping platforms or imputation [3] , [4] based on previous releases of the HapMap [5] and the 1,000 Genomes pilot projects [6] . The latest release (phase 1) of the 1,000 Genomes Project (1,000G) haplotypes consists of 39.7 million genetic markers including 1.4 million indels. By applying genotype imputation techniques [3] , [4] on this high-quality reference panel from 1,000G (ref. 7 ), we can assess the genetic effect of indels as well as low-frequency SNPs on disease phenotypes and gene expression. Indels are the second-most abundant category of genetic variants and are widely distributed in the human genome. Comparing with SNPs, it is still unknown whether this type of structural variant has a larger causal effect on traits of interest, or serves as better tags of the causal genetic variants. A recent study based on 179 sequenced samples from the 1,000G has shown that indels are generally subject to stronger purifying selection than SNPs and they are enriched in associations with gene expression [8] . Imputation of these newly identified genetic variants into existing GWAS may help identifying novel disease loci not discovered by previous genotyping platforms and imputation. But it is not known how much unidentified disease heritability is due to indels and to what extent previously identified disease-associated SNPs are due to linkage disequilibrium with indels of bigger impact on disease phenotype. Interindividual variation in gene expression levels has a significant heritable component [9] , [10] , [11] , [12] , [13] , and studies have mapped individual genetic variants associated with gene expression levels, known as expression quantitative trait locus (eQTL), in diverse cell types [9] , [14] , [15] , [16] , [17] , [18] , [19] , [20] . Large-scale gene expression data, which provide complex traits with full spectrum of heritability and genetic architecture, is ideal for evaluation of the power of association study using imputation of the newly identified indels. This information will be useful to the research community as to what should be expected from the imputation of indels and guide the design of genotyping platforms for the next-generation association studies. Functional annotations generated from eQTL mapping, most of which available to the public, is an important resource to interpret variants of human genome [21] . It is well known that eQTLs can be a useful tool to characterize the function of a disease-associated variant and point to the underlying biological pathways [22] , [23] , [24] , [25] , [26] , [27] , [28] , [29] , [30] , [31] , [32] , [33] , [34] , [35] , [36] , [37] , [38] , [39] , [40] , [41] , [42] , [43] , [44] , [45] , [46] , [47] . With the available 1,000G indel reference panel, existing GWAS are doing imputation on these indels. Once disease-associated indels are identified, their functional interpretation will become essential. We expect that indel eQTL will be a useful tool to characterize the findings of GWAS based on indels, either by imputation or genotyping experiments. Tissue-specific effects of small insertions and deletions on gene expression have not been examined before. Whether the tissue specificity of eQTL effects shows different patterns in SNPs and structure variants is unknown. In this study, we use 1,000G imputed indels from 718 samples of multiple tissue types to answer the above questions and discussed their implication for disease mapping studies. It helps to understand the underlying genetic architecture of gene expression across tissues and interpret the function of disease- and trait-associated structure variants. Indel imputation We collected tissue gene expression data from three studies: (1) gene expression in lymphoblastoid cell lines (LCLs) from the MRCA family panel of 206 siblings of British descent [13] . A total of 368 children were genotyped using the Illumina Sentrix HumanHap300 BeadChip (ILMN300K) and the Illumina Sentrix Human-1 Genotyping BeadChip (ILMN100K); (2) gene expression in peripheral blood mononuclear cells (PBMC) from 47 Germany eczema nuclear families [48] . A total of 240 individuals (107 children, 133 parents) were genotyped using Affy500K and Affy 6.0 SNP array; and (3) normal skin tissues of 57 unrelated healthy controls and unaffected skin of 53 patients from a Psoriasis GWAS [49] . A total of 110 individuals were genotyped with Perlegen 400K array. Gene expression was measured using the Affymetrix HG-U133 Plus 2.0 GeneChip. After quality control on genotypes and expression, 376,877 SNPs from the LCL expression data set, 687,364 from the PBMC expression data set, 433,964 from the skin expression data set, as well as 51,190 gene expression probe sets remain for downstream analysis (see Methods section for details). A total of 39.7 million genetic markers including 1.4 million indels from the phase 1 release of 1,000G (ref. 7 ) were imputed [3] into these three data sets, separately. Among these variants, 814,715 indels and 10,129,531 SNPs have high-quality score (imputation R 2 >0.3 in all three studies). Across the entire allele frequency spectrum, indel imputation quality was generally comparable to that of SNPs but showed a slightly smaller fraction with extremely high imputation score ( R 2 >0.95, for common variants, Supplementary Fig. 1 ). Imputation quality for both SNPs and indels were similar across studies based on different genotype platforms (Pearson correlation between quality score (MACH Rsq) from PBMC and skin data sets were 0.727 (SNP) and 0.811 (indel); 0.696 (SNP) and 0.786 (indel) between PBMC and LCL data sets; 0.736 (SNP) and 0.814 (indel) between LCL and skin data sets). All downstream analyses were based on SNPs and indels with imputation quality R 2 >0.3 across all three studies. eQTL meta-analysis Within each individual study, we tested for association between the gene expression and imputed SNPs and indels using MERLIN package [50] , [51] accounting for family relatedness and including sex and expression principal components in the model [52] . The number of expression principal components was chosen to maximize the number of transcription probes that can be mapped by a variant within 1 Mb of the probe set with false discovery rate (FDR)<5%. Results from individual studies were then combined using weighted Z -score meta-analysis with sample size and imputation R 2 as weights. We corrected for multiple testing using the Benjamini–Hochberg FDR [53] , [54] accounting for all probe set-variant pairs ((814,715 indel+10129531 SNP)*51190 probe set). At FDR<5%, a total of 5,898 unique genes (corresponding to 10,364 unique probe sets) were mapped by both SNP and indel; 325 unique genes (428 unique probe sets) can only be mapped by indels and 3,186 unique genes (6,663 unique probe sets) can only be mapped by SNPs ( Fig. 1a ). Of the 9,409 genes mapped by SNPs or indels or both, 3,024 (32.1%) genes have indel as the most significant eQTL. We summarized our results based on the eQTLs that passed the>5% FDR threshold. For genes that have both significant SNP and indel, the heritability explained by the eQTL is apparently larger than the genes mapped by only SNP or indel ( Fig. 1b ). 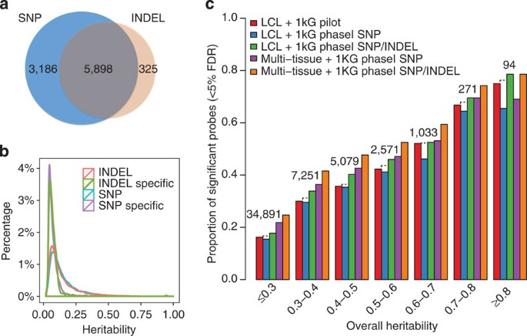Figure 1 Meta-analysis result for association between gene expression and imputed indels and SNPs. (a) Venn diagram for unique number of genes only mapped by SNP or indel or both. (b) Density curve of heritability of gene expression (H2) explained by the top SNP and indel. Red:H2of the top indel for the 5,898 genes ina. Green:H2of the top indel for the 325 genes ina. Blue:H2of the top SNP for the 5,898 genes ina. Purple:H2of the top SNP for the 3,186 genes ina. (c) Per cent of probes mapped by eQTL (<5% FDR) by total narrow-sense heritability for 51,190 transcription probes. Probes were categorized by total narrow-sense heritability previously estimated based on the MRCA family panel. The red bar shows the per cent of probes mapped by eQTL using the MRCA LCL data alone with imputation of the 1,000G pilot releases. The blue bar shows the per cent of probes mapped using imputation of 1,000G phase 1 variants in MRCA data set excluding probes with indel as the top eQTL. The dash box on top of the blue bar indicates the per cent of mapped probes before excluding probes with indel as top eQTL. The green bar shows the per cent of probes mapped using imputation of 1,000G phase 1 variants in the MRCA data set. The purple bar shows the per cent of probes mapped using meta-analysis across three tissues excluding the probes with indel as the top associated variants. The orange bar shows the per cent of probes mapped using meta-analysis across three tissues. The numbers on top of each group of bars are the number of probes in each heritability category. Figure 1 Meta-analysis result for association between gene expression and imputed indels and SNPs. ( a ) Venn diagram for unique number of genes only mapped by SNP or indel or both. ( b ) Density curve of heritability of gene expression ( H 2 ) explained by the top SNP and indel. Red: H 2 of the top indel for the 5,898 genes in a . Green: H 2 of the top indel for the 325 genes in a . Blue: H 2 of the top SNP for the 5,898 genes in a . Purple: H 2 of the top SNP for the 3,186 genes in a . ( c ) Per cent of probes mapped by eQTL (<5% FDR) by total narrow-sense heritability for 51,190 transcription probes. Probes were categorized by total narrow-sense heritability previously estimated based on the MRCA family panel. The red bar shows the per cent of probes mapped by eQTL using the MRCA LCL data alone with imputation of the 1,000G pilot releases. The blue bar shows the per cent of probes mapped using imputation of 1,000G phase 1 variants in MRCA data set excluding probes with indel as the top eQTL. The dash box on top of the blue bar indicates the per cent of mapped probes before excluding probes with indel as top eQTL. The green bar shows the per cent of probes mapped using imputation of 1,000G phase 1 variants in the MRCA data set. The purple bar shows the per cent of probes mapped using meta-analysis across three tissues excluding the probes with indel as the top associated variants. The orange bar shows the per cent of probes mapped using meta-analysis across three tissues. The numbers on top of each group of bars are the number of probes in each heritability category. Full size image Previous studies have shown that the power to detect eQTL increases with total additive heritability of gene expression estimated from pedigree data [13] . In Fig. 1c , we compared the power to detect association (FDR<5%) across different strategies. The overall heritability is the narrow-sense heritability estimated based on previous study using the MRCA family panel [52] . Within each heritability bin, the red bar shows the per cent of expression probes mapped by using the MRCA LCL data alone with imputation of the 1,000G pilot release (eight million SNPs). Using the same MRCA sample but with imputation of the 1,000G phase 1 SNPs and indels (green bars), we observed that 9.90% more probes were mapped at the same FDR (green versus red bars). By combining the results from multiple tissues, we observed that 41.9% more probe sets can be mapped by at least one genetic variant (orange versus red bars). Disease- or trait-associated genetic variants identified from GWAS were usually not the causal variants but markers in linkage disequilibrium with the causal variants. Almost all GWAS used SNPs as genetic markers to tag underlying causal genetic variants of the disease or trait of interest. By contracting the results based on different imputation strategies, we estimated how many previously identified associations might be tagging the association between the trait and indel. The blue bar in Fig. 1c shows the per cent of probes mapped by 1,000G phase 1 SNPs after removing the probes with indel as the top eQTL. Comparing the red and the blue bars, we found that 3.62% of previously identified SNP QTL (eSNP) in LCL were likely to be tagging the indel eQTL (eindel) of the same gene in LCL. The dash bar on top of the blue bar shows the per cent of probes mapped by 1,000G phase 1 SNPs before removing the probes with indel as the top eQTL, indicating a small gain of power by using the phase 1 SNPs. After combining multiple tissues to increase sample size, this difference increased to 9.20% (purple versus orange) indicating that indels are more likely to be the causal genetic variants for these genes. Comparison of SNP and indel eQTLs To better understand the eQTLs due to SNP and indel effect, we sought to characterize the difference in indel eQTL and SNP eQTL by effect size, allele frequency spectrum and genomic distribution. We first tested whether indels were enriched with eQTL by randomly selecting 100,000 SNP and 100,000 indel with high imputation quality ( R 2 >0.3) from the 1000 Genomes reference. There were 7,987 eSNPs and 11,386 eindels in the selected set of SNPs and indels. The enrichment of eQTLs in indels was significantly more than among SNPs ( χ 2 -test for homogeneity, P value<2.2*10 −16 ). Of the 5,898 genes mapped by both SNPs and indel that passed the 5% FDR threshold, the effect size ( H 2 explained by the variant) of eindel was similar to eSNP (mean difference=−0.007, s.d.=0.048, Fig. 2a ). 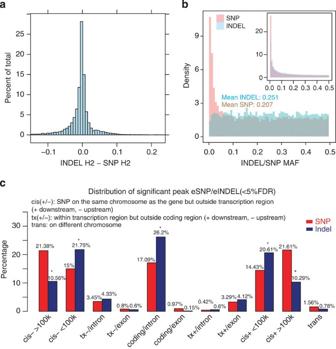Figure 2 Comparison of eSNP and eindel. (a) Histogram of the effect size (heritability explained by the individual eSNP or eindel) difference between eindel and eSNP. (b) Histogram of MAF for eindel (blue) and eSNP (red). Top right small histogram shows MAF distribution for all indel (blue) and SNP (red) with good imputation quality (R2>0.3). (c) Genomic distribution of peak eQTLs (cisortrans) related to the associated gene. For a particular SNP-probe pair or indel-probe pair, we divided the genome into 11 regions related to the gene: upstream TSS >100 kb (cis− >100 k), upstream TSS <100 kb (cis− <100 k), intron between TSS and translation start sites (tx−/intron), exon between TSS and translation start sites (tx−/exon), intron in translation region (coding/intron), exon in translation region (coding/exon), intron between translation stop sites and TES (tx+/intron), exon between translation stop sites and TES (tx+/exon), downstream of TES <100 kb (cis+ <100 k), the downstream TES >100 kb (cis+ >100 k) and on different chromosomes (trans). We then assigned the peak eSNP or eindel into one of these categories, respectively, for SNP and indel, and reported the percentage of total peak eSNP or eindel fell into each category. A star on the top of bar indicates significant difference between eSNP and eindel (P<10−4). Figure 2 Comparison of eSNP and eindel. ( a ) Histogram of the effect size (heritability explained by the individual eSNP or eindel) difference between eindel and eSNP. ( b ) Histogram of MAF for eindel (blue) and eSNP (red). Top right small histogram shows MAF distribution for all indel (blue) and SNP (red) with good imputation quality ( R 2 >0.3). ( c ) Genomic distribution of peak eQTLs ( cis or trans ) related to the associated gene. For a particular SNP-probe pair or indel-probe pair, we divided the genome into 11 regions related to the gene: upstream TSS >100 kb ( cis − >100 k), upstream TSS <100 kb ( cis − <100 k), intron between TSS and translation start sites (tx−/intron), exon between TSS and translation start sites (tx−/exon), intron in translation region (coding/intron), exon in translation region (coding/exon), intron between translation stop sites and TES (tx+/intron), exon between translation stop sites and TES (tx+/exon), downstream of TES <100 kb ( cis + <100 k), the downstream TES >100 kb ( cis + >100 k) and on different chromosomes ( trans ). We then assigned the peak eSNP or eindel into one of these categories, respectively, for SNP and indel, and reported the percentage of total peak eSNP or eindel fell into each category. A star on the top of bar indicates significant difference between eSNP and eindel ( P <10 −4 ). Full size image Among all eSNPs and eindels that passed 5% FDR, allele frequency of eindels were higher than eSNPs (mean minor allele frequency (MAF) of eindel=0.25, mean MAF of eSNP=0.21, Fig. 2b , main panel). This difference is not due to the distribution of SNPs and indels with good imputation quality, where most low-frequency indels were not eQTL ( Fig. 2b , small panel). Next we examined the genomic distribution of eSNPs and eindels by focusing on the peak eQTL (either SNP or indel, cis or trans ) for each probe set with at least one significant eQTL (5% FDR) and divided the genome into 11 regions: upstream TSS >100 kb ( cis − >100 k), upstream TSS <100 kb ( cis − <100 k), intron between TSS and translation start sites (tx−/intron), exon between TSS and translation start sites (tx−/exon), intron in translation region(coding/intron), exon in translation region (coding/exon), intron between translation stop sites and TES (tx+/intron), exon between translation stop sites and TES (tx+/exon), downstream of TES <100 kb ( cis + <100 k), the downstream TES >100 kb ( cis + >100 k) and on different chromosomes ( trans ). We found that eindels were significantly enriched in intron in translation region, upstream 5′ untranslated region, UTR ( cis − <100 k) and downstream 3′UTR ( cis + <100 k) of the associated gene, and were depleted in exon, distal cis effect ( cis − >100 k and cis + >100 k, Fig. 2c ). This pattern did not change after restricting to common SNPs and indels. ( Supplementary Fig. 2a ) and eindels seem to show larger effect size and more significant evidence (larger LOD score) than eSNPs in these three regions ( Supplementary Fig. 2b,c ). Except for the well-known depletion of indel in exons [7] , the enrichment and depletion in other regions cannot be explained by genomic distribution of available SNPs and indels with high imputation quality ( Supplementary Data 1 ). We hypothesized that eindels are more likely to be causal eQTLs in intron in translation region and regions close to 5′ and 3′UTR, but this remains to be confirmed by experiments. Tissue-specific eQTLs For a particular SNP-probe set pair, the eQTL effect may present (coded as 1) in a particular tissue or not (coded as 0). For the three tissues we studied, this resulted in eight possible scenarios (from not being an eQTL in any tissues 000 to being eQTL in all the three tissues 111, corresponding to the order of LCL, PBMC and SKIN). We investigated tissue-specific eQTL effects for each SNP-probe set pair by estimating the posterior probability of each of the eight possible scenarios (see Methods for detail). We denoted P 111 as the posterior probability that the eQTL effect presented in all three tissues and P tissue-specific eQTL (tse) =1− P 000 − P 111 as the probability that eQTL effect presented in at least one but not all tissues. We found that for cis eQTLs (defined as SNP/indel and probe set are within 1 Mb of each other), the mean of P tse across all 930,775 SNP-probe set pairs from meta-analysis (<5% FDR) were 0.448 (s.d. 0.369), the mean of P 111 were 0.552 (s.d. 0.369) and the mean of P 000 was 6.15 × 10 −5 . This suggests that cis eQTLs are more likely to be shared between tissues but still many were tissue specific. On the contrary, the mean P tse for trans eQTLs (defined as SNP and probe set being either on different chromosomes or >500 kb apart) was 0.806 (s.d. 0.121) and the mean of P 111 was 0.192 (s.d. 0.121; Supplementary Fig. 3a–d ). Results for eindels were similar ( Supplementary Fig. 3 e-h ). This clearly showed that trans eQTLs are much less likely to be shared between tissues. Genes with shared genetic regulators across tissues might have different functions than genes with tissue-specific regulators. Characterizing gene pathways and functional groups by tissue sharing of genetic regulators would help understand the underlying regulation of such pathways and help prioritizing genetic studies using related tissues. We used gene ontology (GO) biological process to characterize the functions of genes based on annotation information downloaded from the manufacture’s website. For each scenario of eQTL sharing (P 000 , …, P 111 ), both Z -score and permutation-based P values were used to assess significance. For each GO category, we focused on the peak eQTL on the same chromosome of the probes belonging to genes in this category. We then asked whether eQTLs for this GO category showed significant high level of posterior probability for each of the eight sharing scenarios, respectively. Accounting for 199 GO terms (number of genes >20) and a 5% family-wise false-positive rate, the Bonferroni correction gave a significant P value threshold of 2.5 × 10 −4 ( Supplementary Table 2 ). We found that genetic regulators for genes involved in ‘translation’ ( P <1.62 × 10 −5 ), ‘oxidation–reduction’ ( P <1.65 × 10 −4 ) and ‘proton transport’ ( P <2.89 × 10 −4 ) were likely shared between all three tissues ( P 111 ). Genes involved in ‘response to protein stimulus’ ( P <6.57 × 10 −7 ) were likely sharing similar genetic regulation in PBMC and skin ( P 011 ). Genes involved in ‘oxidation–reduction’ ( P <2.29 × 10 −7 ) and ‘metabolic process’ ( P <4.18 × 10 −6 ) were likely sharing similar genetic regulation in LCL and skin ( P 101 ). ‘tRNA processing’ ( P <6.30 × 10 −4 ) were marginal significantly shared between LCL and PBMC ( P 110 ; Supplementary Data 2 ). Potential epigenetic driving factors for eQTLs Genetic regulatory variants may affect the gene expression level by different functional mechanisms. To identify the potential functional role of eQTLs, functional elements predicted by using ENCODE data were downloaded from UCSC genome browser (hg19) [55] . We pooled the annotation data from the tracks for skin (NHEK) and blood (GM12878) for mapping and analysis of chromatin state dynamics of peak eQTLs (either eSNPs or eindels in cis or trans ) identified from this study. This strategy has been shown to be a powerful way to interpret the function of eQTLs and generate specific hypothesis for gene expression regulation, as demonstrated in the Crohn’s disease and PEGER4 gene eQTL example [56] . We divided the peak eSNPs and eindels into three groups according toMAF: MAF<0.05, 0.05≤MAF<0.10 and 0.10≤MAF≤0.50, and examined the overlap with each available functional element. Across all three MAF groups, we found that both types of eQTLs (eSNP and eindel) were significantly enriched ( P value<10 −4 by permutation test comparing with MAF-matched and distance-to-gene-matched SNPs and indels chosen from 1,000G) in functional elements, including active promoter, weak promoter, transcriptional elongation and weak transcribed ( Fig. 3b–d ). They were both significantly depleted in heterochromatin marks ( Fig. 3a ). Both types of eQTLs showed non-significant overlap with functional elements for inactive/poised promoter, insulator, polycomb-repressed and common copy-number variation ( Fig. 3b-d ), and were marginally significant for rare CNVs ( P =0.0012 for both eSNP and eindel). For strong enhancer and weak/poised enhancer, common eQTLs were enriched in these two functional elements while rare eQTLs were marginally significantly enriched ( P ranges from 0.0011 to 0.0015). Finally, for transcriptional transition, both common and low-frequent eindels were enriched but only common eSNPs (MAF>5%) were enriched in this functional element (rare eSNP P value=0.58). To compare between indels and SNPs, we found that transcriptional elongation and weak transcribed were significant different between indels and SNPs ( P value<1 × 10 −4 ). Active promoter was significantly different in common eSNPs (MAF>5%; P value<1 × 10 −4 ). Transcriptional transition was significantly different in rare eSNPs (MAF<10%; P value<1 × 10 −4 ). P value was calculated using simulation by randomly selected SNPs or indels from the same MAF category and genome within ±500 Kb of any genes. These functional annotations for individual peak eQTLs that passed the 5% FDR threshold are available in Supplementary Data 3 . Association results (effect size, LOD score, P value and so on) for these eQTLs were also provided in this table. 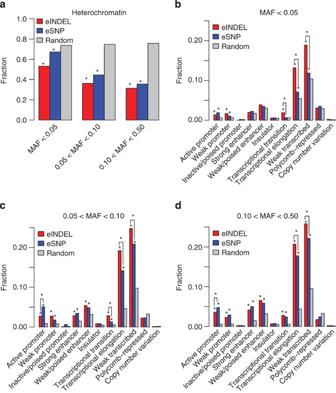Figure 3 Distribution of peak eQTLs in functional regulator elements based on ENCODE data. (a) The fraction of eindel (red bars) and eindel (blue bars) within heterochromatin marks (Ernstet al.55) by different ranges of MAF (MAF<0.05, 0.05≤MAF<0.1, 0.1≤MAF≤0.5). A star on the top of bar indicates significant depletion (P<10−4, Bonferroni correction for 12 × 3 categories is 0.05/36=1.39 × 10−3). (b–d) The fraction of eindel (red bars) and eindel (blue bars) in functional elements (Ernstet al55) by different ranges of MAF (b: MAF<0.05,c: 0.05≤MAF<0.1,d: 0.1≤MAF≤0.5) compared with randomly selected SNPs from the same MAF category and genome within ±500 kb of any genes (grey colour). Statistically different between eindels and eSNPs are also compared. A star on the top of bar indicates significant enrichment (P<10−4, Bonferroni correction for 12 × 3 categories is 0.05/36=1.39 × 10−3). A star with solid lines connecting the SNP and indel bars indicates significant difference between the SNP and indel categories (P<10−4). Figure 3 Distribution of peak eQTLs in functional regulator elements based on ENCODE data. ( a ) The fraction of eindel (red bars) and eindel (blue bars) within heterochromatin marks (Ernst et al . [55] ) by different ranges of MAF (MAF<0.05, 0.05≤MAF<0.1, 0.1≤MAF≤0.5). A star on the top of bar indicates significant depletion ( P <10 −4 , Bonferroni correction for 12 × 3 categories is 0.05/36=1.39 × 10 −3 ). ( b – d ) The fraction of eindel (red bars) and eindel (blue bars) in functional elements (Ernst et al [55] ) by different ranges of MAF ( b : MAF<0.05, c : 0.05≤MAF<0.1, d : 0.1≤MAF≤0.5) compared with randomly selected SNPs from the same MAF category and genome within ±500 kb of any genes (grey colour). Statistically different between eindels and eSNPs are also compared. A star on the top of bar indicates significant enrichment ( P <10 −4 , Bonferroni correction for 12 × 3 categories is 0.05/36=1.39 × 10 −3 ). A star with solid lines connecting the SNP and indel bars indicates significant difference between the SNP and indel categories ( P <10 −4 ). Full size image Comparison of eQTLs with known GWAS loci SNP eQTLs have been widely used to characterize the function of a disease-associated variant and point to the underlying biological pathways [22] , [23] , [24] , [25] , [26] , [27] , [28] , [29] , [30] , [31] , [32] , [33] , [34] , [35] , [36] , [37] , [38] , [39] , [40] , [41] , [42] , [43] , [44] , [45] , [46] , [47] . The newly identified eSNPs and in particular eindels may continue to help interpret the function of GWAS loci that could not be explained before. We examined the disease- and trait-associated loci from the NHGRI GWAS category (downloaded from http://www.genome.gov/GWAStudies/ on 15 March 2013). Considering the diseases and traits with more than 10 reported genes ( Supplementary Table 4 ) and all cis and trans eQTLs that passed the 5% FDR threshold, we found that top diseases or traits enriching genes with significant eSNPs include mean corpuscular haemoglobin concentration, response to amphetamines and red blood cell count, while top diseases or traits enriching genes with significant eindelS include tonometry, IgE levels, mean corpuscular haemoglobin concentration, coeliac disease and rheumatoid arthritis. We also examined tissue-specific eQTLs among GWAS variants and found that tonometry was among the top list with ⩾ 50% trait-associated genes were regulated by tissue-specific eindels, while temperament (bipolar disorder), adiponectin levels and glycated haemoglobin levels were among the top list with ⩾ 60% disease or trait-associated genes regulated by tissue-specific eSNPs ( Supplementary Data 4 ). This is the first study to impute short insertion and deletion (indel) genome-wide in eQTL mapping study, which provided unique opportunities to answer several important questions. Our results suggested that imputation of indels can increase the power of GWAS for complex traits by about 10%. Although this was an estimate based on gene expression traits with complex genetic architecture and full spectrum of heritability, the power gain for particular disease or traits would vary by their specific genetic background. After the completion of the 1,000G, many more high-quality indels will be available for imputation and the reference panel will be increased from the current 1,092 to 2,500 subjects. We expected that the power gain by imputation of indel will be even larger. Our results also suggested that a substantial fraction of previous identified disease- and trait-associated SNPs were markers in linkage disequilibrium of indels with larger effect. Imputation of indels into GWAS would help fine map the causal variants that were tagged by previous studies. As seen in our study, this fraction of SNPs tagged by indel would increase as power increases. In our case, it increases from 3.62 to 9.20% as sample size increases from 368 to 718. Previous studies and this study has shown that SNP eQTLs were enriched in intron and regions closed to UTRs; our study is the first one to show that indel eQTLs were even more enriched in these three regions (defined as intron in translation region, 100 kb upstream of 5′ UTR and 100 kb of downstream of 3′ UTR). We hypothesized that this is because indel is more likely to be causal regulator as they are more likely to destruct splice sites and promoter regions but further experiments are required to validate these hypotheses. Finally, this study showed that cis eQTLs were more likely to be shared across tissues, while trans eQTLs were more likely to be tissue specific. This is consistent with previous findings [10] . Indel eQTLs and SNP eQTLs showed similar pattern for tissue specificity for cis and trans . It suggested that the tissue-differentiated genetic regulation is not related to the size of the genetic variants. All significant SNP and indel eQTLs identified from this study are freely accessible to the public. We expect that it will be an important resource for GWAS to interpret function of genetic variants for complex diseases and traits, particular for structure variants. Data resources This study includes data from three former studies: (1) MRCA contained 206 siblings of British descent [13] . A total of 368 children were genotyped using the Illumina Sentrix HumanHap300 BeadChip (ILMN300K) or the Illumina Sentrix Human-1 Genotyping BeadChip (ILMN100K) or both. Global gene expression in LCLs was measured using Affymetrix HG-U133 Plus 2.0 GeneChip (including 54,675 transcript probes). (2) Two hundred and forty individuals from 47 Germany eczama families were genotyped with Affy500K and Affy 6.0 SNP array. The gene expression level of their PBMC was evaluated with Affymetrix U133 Plus 2.0 GeneChip. (3) Normal skin tissues of 110 subjects from a former Psoriasis GWAS were genotyped with Perlegen 400K array and the RNA expression level was evaluated with the same Affymetrix GeneChip. 3,423 probe set which can be mapped to multiple genome position (based on HG-U133 Plus_2 annotations file, release 34) and 62 Affymetrix control probes were removed in our analysis. SNP quality control and imputation SNPs were excluded from further analysis with the following criteria: (1) the SNP has more than two alleles; (2) the SNP is not presented in the 1,000G phase 1 release; (3) the SNPs were genotyped in <95% samples; (4) the Hardy–Weinberg test is significant with P value<10 −6 ; (5) the MAF of the SNP <0.01. SNPs and indels from the 1,000G phase 1 release (2012-03-14 haplotypes) were imputed using MINIMAC [57] . A total of 814,715 indels and 10,129,531 SNPs had high-quality score ( R 2 >0.3 in three studies). Meta-analysis We used a weighted z -score in meta-analysis. To account for different imputation qualities and sample sizes in the three studies, we used a weighted scheme: and here the weight is a combination of sample size and imputation quality: , where is as defined in Li et al . [3] To control for multiple testing, a cutoff of FDR<0.05 accounting for all SNP/indel-probe set pairs were used, corresponding to a P value of <2.58 × 10 −6 . Inference of tissue-specific effect Following Wakefield [58] , we used y to denote the observed data and H 1 the alternative hypothesis, then for the quantitative trait: y = x T γ + Zθ , where β =( γ , θ ) are parameters corresponding to the effects of covariates x and SNP z . According to Wakefield [58] , when calculating asymptotic Bayesian factor (ABF), we only need to consider the sampling distribution of the MLE: and the prior for θ ∼ N ( 0 , W ), which gives: An advantage of using ABF is that the calculation only involves and its s.e. from individual studies. And from the above we can calculate ABF 1 , ABF 2 and ABF 3 for the three tissues, respectively. We defined all possible scenarios for tissue sharing as in Table 1 . Then the posterior probability of each scenario can be calculated. Table 1 Definition of all different tissue-specific eQTLs. Full size table We defined probability of being tissue-specific eQTL ( P tse ) as: Here P 111 is the posterior probability of sharing eQTLs across all three tissues, while P 000 is the probability that the eQTL does not occur in any tissue. Bayesian factor for each scenario in Table 1 can be computed based on Bayesian factors from individual studies, for example, BF c1 is given in formula. Then the posterior probability of P 111 is calculated as: , assuming equal prior probabilities π i =1/8, i =000 to 111. The posterior probability of the other seven scenarios can be computed in a similar way. GO enrichment analysis The Affymetrix expression probes were grouped into GO categories using annotation information downloaded from the manufacturer’s website. For each GO category, we focused on the peak eQTL (FDR<5%) on the same chromosome of the probes belonging to genes in this category and calculated the mean of P(000), …, P(111) of these eQTLs, denoted as G i for the i th GO category for each of the eight scenarios, respectively. The Z -score for the ith GO category is , where μ is the overall mean of P(000), …, P(111) for all probes annotated to the 9,409 genes, respectively, σ is the corresponding s.d. and n i is the number of probes for the ith GO category that mapped by eQTL. The P value is computed by comparing the Z -score with a standard normal distribution for one-sided test. We also computed the permutation-based P value by shuffling the correspondence between probes and GO categories while maintaining the same number of genes for each GO term. From 10,000 permutations, we counted how many times ( M i ) the G i based on permutated data were larger than G i based on observed data. The permutation-based P value is M i /10,000. Genomic distribution of SNP and indel eQTLs Genome annotation was obtained from the UCSC genome browser (hg19). To examine the distribution of the physical location of cis and trans eSNPs and eindels, we focused on peak eQTLs ( cis or trans ) for each probe set. For a particular SNP-probe pair or indel-probe pair, we divided the genome into 11 regions related to the gene: upstream TSS >100 kb ( cis − >100 k), upstream TSS <100 kb ( cis − <100 k), intron between TSS and translation start sites (tx−/intron), exon between TSS and translation start sites (tx−/exon), intron in translation region (coding/intron), exon in translation region (coding/exon), intron between translation stop sites and TES (tx+/intron), exon between translation stop sites and TES (tx+/exon), downstream of TES <100 kb ( cis + <100 k), the downstream TES >100 kb ( cis + >100 k) and on different chromosomes ( trans ). We then assigned the peak eSNP or eindel into one of these categories, respectively, for SNP and indel, and reported the percentage of peak eSNP or eindel fell into each category. Distribution of SNP and indel eQTLs related to epigenetic factors Functional elements predicted by using ENCODE data were downloaded from UCSC genome browser (hg19) [55] . We pooled the data from the skin (NHEK) and blood (GM12878) tracks for mapping and analysis of chromatin state dynamics. SNPs and indels located within these functional elements were considered as related to epigenetic factors. For this analysis, we focused on peak eQTLs (either eSNPs or eindels in cis or trans ). For each MAF category (MAF≤0.05, 0.05<MAF≤0.1, 0.1<MAF≤0.5), we calculated the fraction of eSNPs or eindels fell into each functional element category. The significance of enrichment was determined by randomly selecting the same number of SNPs or indels from the same MAF category and computed the fraction of random SNPs or indels fell into these functional regulatory regions. We counted how many times ( M ) the fraction of random SNP or indel as larger than the fraction based on eSNPs or eindels. Enrichment P value ( Fig. 3b-d ) was calculated as M /10,000 for 10,000 permutations. Depletion P value ( Fig. 3a ) was calculated as 1− M /10,000. Overlapping with known GWAS-reported genes GWAS results were obtained from the NHGRI GWAS database (downloaded from http://www.genome.gov/admin/gwascatalog.txt on 10 January 2014). GWAS-reported genes were obtained from the ‘Reported Gene’ column in gwascatalog.txt file. For each disease or trait, we calculated the per cent of reported genes associated with at least one SNP or indel, respectively. We also calculated the percentage of reported genes associated with eSNP or eindel that showed tissue-specific effects ( P tse >0.5) Online resources On our website ( http://eqtl.rc.fas.harvard.edu/indeleQTL/ ), we provided flat tables (csv files) for all eQTL results with meta-analysis FDR<0.05. How to cite this article: Huang, J. et al . eQTL mapping identifies insertion and deletion specific eQTLs in multiple tissues. Nat. Commun. 6:6821 doi: 10.1038/ncomms7821 (2015).